Filamin acts as a key regulator in epithelial defence against transformed cells Recent studies have shown that certain types of transformed cells are extruded from an epithelial monolayer. However, it is not known whether and how neighbouring normal cells play an active role in this process. In this study, we demonstrate that filamin A and vimentin accumulate in normal cells specifically at the interface with Src- or RasV12-transformed cells. Knockdown of filamin A or vimentin in normal cells profoundly suppresses apical extrusion of the neighbouring transformed cells. In addition, we show in zebrafish embryos that filamin plays a positive role in the elimination of the transformed cells. Furthermore, the Rho/Rho kinase pathway regulates filamin accumulation and filamin acts upstream of vimentin in the apical extrusion. This is the first report demonstrating that normal epithelial cells recognize and actively eliminate neighbouring transformed cells and that filamin is a key mediator in the interaction between normal and transformed epithelial cells. Cell transformation arises from activation of oncoproteins and/or inactivation of tumour suppressor proteins. At the initial stage of carcinogenesis, transformation occurs in single cells within epithelia, and the transformed cells grow while being surrounded by neighbouring normal epithelial cells. In Drosophila , there are a number of reports demonstrating that normal and transformed epithelial cells compete with each other for survival; ‘loser cells’ are extruded from the epithelium or undergo apoptosis, while ‘winner cells’ proliferate and fill the vacant spaces. This process is called ‘cell competition’ [1] , [2] , [3] , [4] , [5] , [6] , [7] , [8] . However, it was not clearly understood what happens at the interface between normal and transformed epithelial cells in vertebrates. Recently, it has been revealed that certain types of transformed cells are extruded from a monolayer of normal cells and leave the epithelium [9] , [10] . For example, we have shown using mammalian cell culture systems that when RasV12-transformed cells are surrounded by normal cells, the RasV12 cells are either apically extruded from the monolayer, or form dynamic basal protrusions and invade the basal matrix [8] . We have also demonstrated that when Src-transformed cells are surrounded by normal cells, Src cells are apically extruded from a monolayer of normal epithelial cells [11] . Apical extrusion of Src-transformed cells is also observed in the outermost epithelium of zebrafish embryos [11] . In addition, ErbB2-overexpressing cells are apically translocated into the lumen of epithelia [12] . These studies shed light on unexplored processes occurring at the initial step of carcinogenesis. Although molecular mechanisms for the apical extrusion of transformed cells are largely unknown, we have shown that various signalling pathways are activated in transformed cells surrounded by normal cells, leading to their extrusions [8] , [11] . For instance, myosin-II and Cdc42 are activated in Ras-transformed cells only when they are surrounded by normal epithelial cells [8] . Similarly, myosin-II, mitogen-activated protein kinase (MAPK) and focal adhesion kinase are activated in Src-transformed cells surrounded by normal cells [11] . Furthermore, inhibition of these signalling pathways substantially suppresses apical extrusion of the transformed cells. These results indicate that modulation of various signalling pathways in transformed cells plays a crucial role in the apical extrusion. However, it is not known whether and how neighbouring normal cells play an active role in the extrusion of transformed cells. Filamin is a homodimeric actin-binding protein that crosslinks and stabilizes cortical F-actin filaments and links them to plasma membranes by binding to transmembrane receptors or ion channels [13] , [14] , [15] , [16] . A V-shape of filamin dimers causes the perpendicular branching of F-actin, generating dynamic orthogonal F-actin networks rather than parallel actin bundles. There are three filamin homologues: filamin A, B and C. Filamin A and filamin B are both ubiquitously expressed, whereas filamin C is specifically expressed in muscles. Filamin A is a large, rod-like protein composed of an amino-terminal actin-binding domain and 24 immunoglobulin (IgG)-like domains. The actin-binding domain and the first 15 IgG-like domains form an elongated structure that binds actin filaments along its length. The16–23 IgG-like domains form more compact, globular structures containing cryptic binding sites that are exposed when the molecule is under tension. The carboxy-terminal IgG-like domain is responsible for dimerization. Filamin binds to numerous proteins, including transmembrane receptors and signalling molecules, and is involved in various cellular processes such as cell adhesion, cell motility and transcriptional control. Moreover, a recent study demonstrated that filamin can also play a role in cellular mechanotransduction [17] . Externally imposed shear stress or myosin-II-driven forces induce deformation of F-actin networks, thereby exposing the cryptic sites of filamin A and modulating its affinity for binding partners. Here, using mammalian cell culture systems, we show that filamin is accumulated in normal epithelial cells at the interface with Src- or Ras-transformed epithelial cells and plays a crucial role in apical extrusion of the transformed cells. Comparable phenomena are also observed in the epithelia of zebrafish embryos. This is the first report demonstrating molecular mechanisms whereby normal epithelial cells actively eliminate neighbouring transformed cells. Filamin A and vimentin identification We have previously shown that when oncogenic v-Src- or RasV12-transformed Madin–Darby canine kidney (MDCK) cells are surrounded by normal MDCK cells, the transformed cells are apically extruded from an epithelial monolayer [8] , [11] . However, when the transformed cells alone are present, they stay in a monolayer, suggesting that the presence of surrounding normal cells induces apical extrusion of the transformed cells. To understand the molecular mechanisms for these phenomena, we have tried to identify molecules that specifically function at the interface between normal and transformed cells. First, cells were cultured under three different conditions: (i) normal MDCK cells alone, (ii) 1:1 mix culture of normal and Src-transformed MDCK cells and (iii) Src-transformed MDCK cells alone. For Src-transformed cells, we used MDCK cells transformed with a temperature-sensitive v-Src mutant (ts-Src MDCK cells) [18] , [19] . We found several molecules that were immunoprecipitated with anti-phospho-tyrosine antibodies predominantly under the mix culture condition ( Fig. 1a ). Among them, using mass spectrometry we identified the 280- and 55-kDa proteins as filamin A and vimentin, respectively ( Fig. 1a , arrow and arrowhead). The identity of these proteins was confirmed by western blotting with anti-filamin or anti-vimentin antibody ( Fig. 1b ). Western blotting with anti-phospho-tyrosine antibody demonstrated that filamin or vimentin per se was not tyrosine phosphorylated, and that vimentin specifically bound to tyrosine-phosphorylated molecules under the mix culture condition ( Supplementary Fig. 1a,b ). Furthermore, the interaction between filamin and vimentin was observed only when normal and Src-transformed cells were co-cultured ( Supplementary Fig. 1c ). These data suggest that the formation of novel protein complexes specifically occurs when normal and transformed epithelial cells interact with each other. 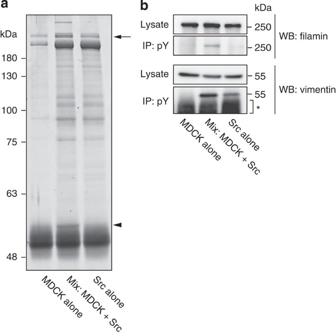Figure 1: Identification of proteins that are specifically modulated when normal and Src-transformed cells interact with each other. (a) SYPRO ruby staining (8% SDS–PAGE) of immunoprecipitated proteins with a mixture of anti-phospho-tyrosine antibodies. The arrow and arrowhead indicate the band for filamin A and vimentin, respectively. (b) Validation of the bands for filamin (upper panels) and vimentin (lower panels) by western blotting. The asterisk indicates heavy chains of IgG. Note that identification or validation of the other bands has not been completed yet. Uncropped scans of immunoblots are shown inSupplementary Fig. 13. Figure 1: Identification of proteins that are specifically modulated when normal and Src-transformed cells interact with each other. ( a ) SYPRO ruby staining (8% SDS–PAGE) of immunoprecipitated proteins with a mixture of anti-phospho-tyrosine antibodies. The arrow and arrowhead indicate the band for filamin A and vimentin, respectively. ( b ) Validation of the bands for filamin (upper panels) and vimentin (lower panels) by western blotting. The asterisk indicates heavy chains of IgG. Note that identification or validation of the other bands has not been completed yet. Uncropped scans of immunoblots are shown in Supplementary Fig. 13 . Full size image Filamin plays an active role in apical extrusion of transformed cells To investigate the function of filamin at the interface between normal and Src-transformed cells, we first examined subcellular localization of filamin by immunofluorescence analysis. We found that filamin was accumulated in the surrounding normal cells at the interface with Src cells ( Fig. 2a,c,d ). When Src activation was not induced, filamin accumulation was not observed ( Fig. 2b,d ). In addition, when Src cells alone were present, filamin accumulation did not occur ( Fig. 2e ). These data indicate that surrounding normal cells recognize the presence of Src-transformed cells and accumulate filamin at the interface. We also found comparable filamin accumulation in normal MDCK cells at the interface with RasV12-transformed MDCK cells ( Fig. 2f ). Filamin was shown to bind orthogonal actin structures, but we did not observe specific actin accumulation in normal cells at the interface with Src-transformed cells ( Supplementary Fig. 2a–c ). However, when F-actin structures were disrupted by cytochalasin D, linear filamin staining pattern was lost ( Fig. 2g and Supplementary Fig. 2d ), suggesting that localization of filamin depends on the intact structure of actin cytoskeletons. To understand the functional involvement of the filamin accumulation in apical extrusion of transformed cells, we established filamin A-knockdown MDCK cells ( Fig. 2h and Supplementary Fig. 3a,b ). Knockdown of filamin A did not affect expression of cell adhesion and cytoskeletal proteins ( Supplementary Fig. 3c ). When Src cells were surrounded by filamin A-knockdown cells, apical extrusion of Src cells was profoundly blocked ( Fig. 2i and Supplementary Fig. 3d ). Similarly, apical extrusion of RasV12-transformed cells was completely blocked when RasV12-transformed cells were surrounded by filamin A-knockdown cells ( Fig. 2j ). These data indicate that filamin A in the surrounding normal cells plays a crucial role in apical extrusion of the transformed cells. 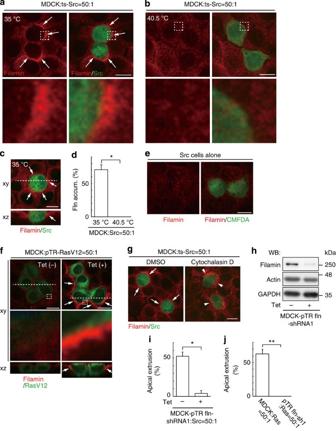Figure 2: Filamin accumulation in the surrounding normal epithelial cells plays a crucial role in apical extrusion of transformed cells. (a–c) Immunofluorescence images of filamin (red) in the mix culture of normal and ts-Src MDCK cells. ts-Src MDCK cells stained with CMFDA (green) were surrounded by normal MDCK cells. v-Src activation was induced at 35 °C (a,c) or not induced at 40.5 °C (b). The area in the white box is shown at higher magnification in the lower panel. Arrows indicate filamin accumulation. (d) Quantification of the filamin accumulation. Data are mean±s.e. from three independent experiments. *P=2.7 × 10−4(Student’st-test). (e) Immunofluorescence images of filamin (red) in the mix culture of Src-transformed cells stained with CMFDA (green) and non-labelled Src-transformed cells. (f) Immunofluorescence images of filamin (red) in the mix culture of normal and RasV12-MDCK cells. RasV12-MDCK cells stained with CMFDA (green) were surrounded by normal MDCK cells. GFP-RasV12 expression was not induced (left panels) or induced by tetracycline (right panels) The area in the white box is shown at higher magnification in the lower panel. Arrows indicate filamin accumulation. White dashed lines inxypanels denote the cross-sections represented inxzpanels (c,f). (g) Effect of cytochalasin D on filamin accumulation in the surrounding normal cells at the interface with Src-transformed cells. ts-Src-MDCK cells stained with CMFDA (green) were mixed with normal cells, and were treated with dimethyl sulphoxide (DMSO) or cytochalasin D followed by immunofluorescence with anti-filamin antibody (red). Arrows or arrowheads indicate intact or disturbed filamin accumulation, respectively. Scale bars, 10 μm (a–c,e–g). (h) Establishment of MDCK cells stably expressing filamin A shRNA1 in a tetracycline-inducible manner. Knockdown was induced for 72 h with tetracycline treatment, followed by western blotting with the indicated antibodies. Note that there are three mammalian filamin homologues (filamin A, B and C), but the majority of filamin proteins in MDCK cells detected by the anti-filamin antibody is filamin A. (i,j) Effect of knockdown of filamin A in the surrounding cells on apical extrusion of Src- (i) or RasV12- (j) transformed cells. Data are mean±s.d. from three (i) or two (j) independent experiments. *P=1.2 × 10−4, **P=0.0031 (Student’st-test). Figure 2: Filamin accumulation in the surrounding normal epithelial cells plays a crucial role in apical extrusion of transformed cells. ( a – c ) Immunofluorescence images of filamin (red) in the mix culture of normal and ts-Src MDCK cells. ts-Src MDCK cells stained with CMFDA (green) were surrounded by normal MDCK cells. v-Src activation was induced at 35 °C ( a , c ) or not induced at 40.5 °C ( b ). The area in the white box is shown at higher magnification in the lower panel. Arrows indicate filamin accumulation. ( d ) Quantification of the filamin accumulation. Data are mean±s.e. from three independent experiments. * P =2.7 × 10 −4 (Student’s t -test). ( e ) Immunofluorescence images of filamin (red) in the mix culture of Src-transformed cells stained with CMFDA (green) and non-labelled Src-transformed cells. ( f ) Immunofluorescence images of filamin (red) in the mix culture of normal and RasV12-MDCK cells. RasV12-MDCK cells stained with CMFDA (green) were surrounded by normal MDCK cells. GFP-RasV12 expression was not induced (left panels) or induced by tetracycline (right panels) The area in the white box is shown at higher magnification in the lower panel. Arrows indicate filamin accumulation. White dashed lines in xy panels denote the cross-sections represented in xz panels ( c , f ). ( g ) Effect of cytochalasin D on filamin accumulation in the surrounding normal cells at the interface with Src-transformed cells. ts-Src-MDCK cells stained with CMFDA (green) were mixed with normal cells, and were treated with dimethyl sulphoxide (DMSO) or cytochalasin D followed by immunofluorescence with anti-filamin antibody (red). Arrows or arrowheads indicate intact or disturbed filamin accumulation, respectively. Scale bars, 10 μm ( a – c , e – g ). ( h ) Establishment of MDCK cells stably expressing filamin A shRNA1 in a tetracycline-inducible manner. Knockdown was induced for 72 h with tetracycline treatment, followed by western blotting with the indicated antibodies. Note that there are three mammalian filamin homologues (filamin A, B and C), but the majority of filamin proteins in MDCK cells detected by the anti-filamin antibody is filamin A. ( i , j ) Effect of knockdown of filamin A in the surrounding cells on apical extrusion of Src- ( i ) or RasV12- ( j ) transformed cells. Data are mean±s.d. from three ( i ) or two ( j ) independent experiments. * P =1.2 × 10 −4 , ** P =0.0031 (Student’s t -test). Full size image Filamin plays a crucial role in apical extrusion in zebrafish embryos Furthermore, we examined whether filamin is involved in apical extrusion of Src-activated cells in vivo . In a previous study, using zebrafish embryos we showed that v-Src-expressing cells were apically extruded from an outermost epithelial monolayer, enveloping layer (EVL) [11] . Using an EVL-specific Gal4-driver line, we have established a zebrafish line expressing green fluorescent protein (GFP) or GFP-filamin A within the EVL epithelium. We found that GFP-filamin A was substantially accumulated at the interface with v-Src-expressing cells ( Fig. 3a ) (54% of 76 v-Src-expressing cells from 16 embryos). In contrast, accumulation of GFP was not observed (0% of 29 v-Src-expressing cells from 7 embryos). Moreover, when expression of filamin A was knocked down by morpholino oligonucleotides, apical extrusion of v-Src-expressing cells was significantly suppressed ( Fig. 3b and Supplementary Fig. 4a,b ), which was rescued by exogenous expression of filamin A ( Fig. 3c and Supplementary Fig. 4c ). These data suggest that filamin is an evolutionarily conserved key regulator in apical extrusion of transformed cells. 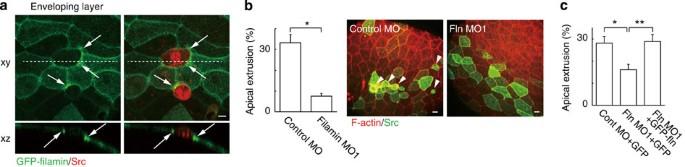Figure 3: Filamin plays a crucial role in apical extrusion of v-Src-expressing cells in the EVL of zebrafish embryos. (a) Confocal images of a GFP-filamin-expressing zebrafish embryo (at 10-11 h post fertilization) expressing v-Src in a mosaic manner. Embryos from an EVL-specific GFP-filamin A-expressing line were injected with the UAS:Cherry-v-Src-expressing vector at the one-cell stage. Arrows indicate GFP-filamin accumulation in the neighbouring EVL cells at the interface with v-Src-expressing EVL cells (red). White dashed lines inxypanels denote the cross-sections represented inxzpanels. (b) Effect of filamin morpholino oligonucleotides (MO) on apical extrusion of v-Src-expressing cells. Embryos were injected with the v-Src-expressing vector and indicated oligonucleotides. Representative images were shown on the right. Arrowheads indicate v-Src-expressing extruded cells. Data are mean±s.e. from ten embryos for control MO and from nine embryos for filamin MO1. *P=1.0 × 10−5(Student’st-test). Scale bars, 10 μm (a), 20 μm (b). (c) Rescue of the effect of filamin MO on apical extrusion by expression of exogenous filamin A. Embryos were injected with the v-Src-expressing vector, indicated oligonucleotides and vector. Note that v-Src and GFP-filamin were specifically expressed in the EVL. Data are mean±s.e. from 12 embryos for control MO+GFP, from 10 embryos for filamin MO1+GFP and from 12 embryos for filamin MO1+GFP-filamin. *P=0.0023, **P=0.0024 (Student’st-test). Figure 3: Filamin plays a crucial role in apical extrusion of v-Src-expressing cells in the EVL of zebrafish embryos. ( a ) Confocal images of a GFP-filamin-expressing zebrafish embryo (at 10-11 h post fertilization) expressing v-Src in a mosaic manner. Embryos from an EVL-specific GFP-filamin A-expressing line were injected with the UAS:Cherry-v-Src-expressing vector at the one-cell stage. Arrows indicate GFP-filamin accumulation in the neighbouring EVL cells at the interface with v-Src-expressing EVL cells (red). White dashed lines in xy panels denote the cross-sections represented in xz panels. ( b ) Effect of filamin morpholino oligonucleotides (MO) on apical extrusion of v-Src-expressing cells. Embryos were injected with the v-Src-expressing vector and indicated oligonucleotides. Representative images were shown on the right. Arrowheads indicate v-Src-expressing extruded cells. Data are mean±s.e. from ten embryos for control MO and from nine embryos for filamin MO1. * P =1.0 × 10 −5 (Student’s t -test). Scale bars, 10 μm ( a ), 20 μm ( b ). ( c ) Rescue of the effect of filamin MO on apical extrusion by expression of exogenous filamin A. Embryos were injected with the v-Src-expressing vector, indicated oligonucleotides and vector. Note that v-Src and GFP-filamin were specifically expressed in the EVL. Data are mean±s.e. from 12 embryos for control MO+GFP, from 10 embryos for filamin MO1+GFP and from 12 embryos for filamin MO1+GFP-filamin. * P =0.0023, ** P =0.0024 (Student’s t -test). Full size image Vimentin in the surrounding cells is involved in apical extrusion Vimentin is one of the intermediate filament proteins and is involved in various cellular processes, such as cell adhesion, cell motility and stress response [20] , [21] , [22] . To understand the function of vimentin at the boundary between normal and Src-transformed cells, we examined subcellular localization of vimentin. We found that vimentin was also accumulated in the surrounding normal cells at the interface with Src cells ( Fig. 4a,c ). When Src activation was not induced, vimentin accumulation was not observed ( Fig. 4b ). To further investigate the interface between normal and Src cells, we performed electron microscopic analyses ( Fig. 4d and Supplementary Fig. 5 ). We found that normal cells produced arm-like extensions as if they held neighbouring Src cells, and that intermediate filament-like structures were abundantly present in these extensions ( Fig. 4d and Supplementary Fig. 5 , arrows). Collectively, these data suggest that normal cells sense the presence of neighbouring Src cells and surround them with intermediate filament-rich protrusions. Next, using MDCK cells stably expressing GFP-vimentin ( Supplementary Fig. 6a ), we analysed the dynamic rearrangement of vimentin filaments during apical extrusion of Src cells. When Src cells were surrounded by GFP-vimentin-expressing cells, GFP-vimentin was accumulated at the interface with Src cells as observed for endogenous vimentin proteins ( Fig. 4e and Supplementary Fig. 6b ). Time-lapse analyses revealed that there were two types of vimentin-rich protrusions that dynamically reacted against Src cells. One was the holding arm-like protrusion that surrounded Src cells ( Fig. 4f , Supplementary Fig. 7a and Supplementary Movie 1 ) and the other was the spiky protrusion that poked Src cells ( Fig. 4g and Supplementary Movie 2 ). These protrusions disappeared after Src cells were apically extruded ( Fig. 4f , Supplementary Fig. 7a and Supplementary Movie 1 ). We also found that holding arm-like vimentin accumulations were often accompanied by the basal extension of the neighbouring Src-transformed cells ( Fig. 4f and Supplementary Fig. 7a–c ). Time-lapse analyses demonstrated that vimentin filaments were accumulated as if they reacted to basal extensions of transformed cells, and that these extensions retracted following the appearance of holding arm-like protrusions, eventually leading to apical extrusion of transformed cells ( Fig. 4f , Supplementary Fig. 7a and Supplementary Movie 1 ). Furthermore, when Src cells were surrounded by vimentin-knockdown cells, apical extrusion and basal extension of Src cells were significantly suppressed and promoted, respectively ( Fig. 5a–c and Supplementary Fig. 8a–d ). In the previous study, we showed that basal protrusion formation of transformed cells suppresses their apical extrusion [8] . Collectively, these data suggest that holding arm-like protrusions positively regulate apical extrusion of transformed cells, at least partially, by suppressing their basal extensions. To further understand the functional role of the vimentin filaments, we examined their mechanical property. When laser irradiation ablated the holding arm-like filaments at the interface with Src cells, the ends of severed filaments were instantly recoiled from each other ( Supplementary Fig. 9a,b and Supplementary Movie 3 ). In contrast, comparable recoiling was not observed for spiky protrusions ( Supplementary Fig. 9c ). These results suggest that holding arm-like vimentin filaments generate contractile forces at the interface that could prevent the neighbouring transformed cells from forming basal extensions and possibly squeeze out the transformed cells (for further discussion on physical property of vimentin filaments, see Supplementary Discussion following Supplementary Fig. 9 ). For RasV12-transformed cells, comparable vimentin accumulation was observed in the surrounding normal cells ( Fig. 5d ), but vimentin-knockdown did not significantly affect apical extrusion of RasV12-transformed cells. As keratin 5/8 was also accumulated at the interface with RasV12-transformed cells ( Fig. 5e ), other intermediate filament proteins may also function at the interface with transformed cells. 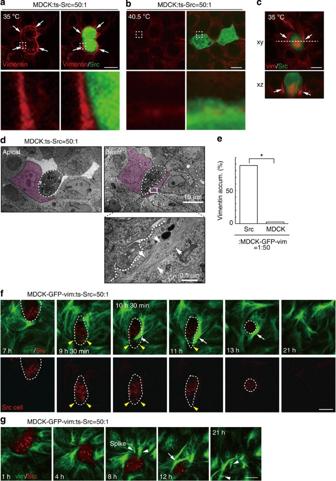Figure 4: Vimentin accumulates in the surrounding normal epithelial cells at the interface with Src-transformed cells. (a–c) Immunofluorescence images of vimentin (red) in the mix culture of normal and ts-Src MDCK cells. ts-Src MDCK cells stained with CMFDA (green) were surrounded by normal MDCK cells. v-Src activation was induced at 35 °C (a,c) or not induced at 40.5 °C (b). The area in the white box is shown at higher magnification in the lower panel. Arrows indicate vimentin accumulation in normal MDCK cells at the interface with ts-Src MDCK cells. The white dashed line in thexypanel denotes the cross-sections represented in thexzpanel (c). (d) Electron microscopic images of the interface between normal and ts-Src MDCK cells. Thexyimages on the apical or basal slice are presented. An Src-transformed cell is traced by the white-dashed line. A purple cell indicates a neighbouring normal cell that produces the specific extension along the Src-transformed cell. The area in the white box is shown at higher magnification in the lower panel. Arrows indicate the accumulation of intermediate filament-like structures. (e) Quantification of GFP-vimentin accumulation around Src-transformed cells using time-lapse microscopy. MDCK GFP-vimentin cells were co-cultured with normal or ts-Src MDCK cells. GFP-vimentin accumulation was analysed for 15 h after the temperature shift. *P=1.6 × 10−30(Fisher’s exact test). (f) Dynamic movements of vimentin-rich protrusions from normal cells towards the neighbouring Src-transformed cells. Images are extracted from a representative time-lapse analysis. ts-Src MDCK cells (stained with CMTPX, red) were mixed with MDCK GFP-vimentin cells. Yellow arrowheads indicate basal extension of a Src-transformed cell. White dashed lines delineate a Src-transformed cell. The presented time in each image indicates the duration of v-Src activation. (g) Dynamic movements of vimentin-rich ‘spiky’ protrusions from normal cells towards the neighbouring Src-transformed cells. Arrows and arrowheads indicate ‘holding arm-like protrusions’ and ‘spiky protrusions’, respectively (f,g). Scale bars, 10 μm (a–c,f,g). Figure 4: Vimentin accumulates in the surrounding normal epithelial cells at the interface with Src-transformed cells. ( a – c ) Immunofluorescence images of vimentin (red) in the mix culture of normal and ts-Src MDCK cells. ts-Src MDCK cells stained with CMFDA (green) were surrounded by normal MDCK cells. v-Src activation was induced at 35 °C ( a , c ) or not induced at 40.5 °C ( b ). The area in the white box is shown at higher magnification in the lower panel. Arrows indicate vimentin accumulation in normal MDCK cells at the interface with ts-Src MDCK cells. The white dashed line in the xy panel denotes the cross-sections represented in the xz panel ( c ). ( d ) Electron microscopic images of the interface between normal and ts-Src MDCK cells. The xy images on the apical or basal slice are presented. An Src-transformed cell is traced by the white-dashed line. A purple cell indicates a neighbouring normal cell that produces the specific extension along the Src-transformed cell. The area in the white box is shown at higher magnification in the lower panel. Arrows indicate the accumulation of intermediate filament-like structures. ( e ) Quantification of GFP-vimentin accumulation around Src-transformed cells using time-lapse microscopy. MDCK GFP-vimentin cells were co-cultured with normal or ts-Src MDCK cells. GFP-vimentin accumulation was analysed for 15 h after the temperature shift. * P =1.6 × 10 −30 (Fisher’s exact test). ( f ) Dynamic movements of vimentin-rich protrusions from normal cells towards the neighbouring Src-transformed cells. Images are extracted from a representative time-lapse analysis. ts-Src MDCK cells (stained with CMTPX, red) were mixed with MDCK GFP-vimentin cells. Yellow arrowheads indicate basal extension of a Src-transformed cell. White dashed lines delineate a Src-transformed cell. The presented time in each image indicates the duration of v-Src activation. ( g ) Dynamic movements of vimentin-rich ‘spiky’ protrusions from normal cells towards the neighbouring Src-transformed cells. Arrows and arrowheads indicate ‘holding arm-like protrusions’ and ‘spiky protrusions’, respectively ( f , g ). Scale bars, 10 μm ( a – c , f , g ). 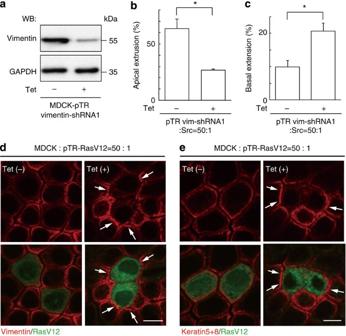Figure 5: Vimentin regulates the fate of Src-transformed cells surrounded by normal epithelial cells. (a) Establishment of MDCK cells stably expressing vimentin shRNA1 in a tetracycline-inducible manner. Knockdown was induced for 72 h with tetracycline treatment, followed by western blotting with the indicated antibodies. (b) Effect of knockdown of vimentin in the surrounding cells on apical extrusion of Src-transformed cells. Data are mean±s.e. from three independent experiments. *P=0.0058 (Student’st-test). (c) Effect of knockdown of vimentin in the surrounding cells on basal extension of Src-transformed cells. Data are mean±s.e. from three independent experiments. *P=0.013 (Student’st-test). (d) Immunofluorescence images of vimentin (red) in the mix culture of normal and RasV12-transformed cells. RasV12-MDCK cells (stained with CMFDA, green) were mixed with normal MDCK cells. (e) Immunofluorescence images of keratin5+8 (red) in the mix culture of normal and RasV12-transformed cells. RasV12-MDCK cells (stained with CMFDA, green) were mixed with normal MDCK cells. Arrows indicate vimentin (d) or keratin5+8 (e) accumulation in normal MDCK cells at the interface with RasV12-MDCK cells. Scale bars, 10 μm (d,e). Full size image Figure 5: Vimentin regulates the fate of Src-transformed cells surrounded by normal epithelial cells. ( a ) Establishment of MDCK cells stably expressing vimentin shRNA1 in a tetracycline-inducible manner. Knockdown was induced for 72 h with tetracycline treatment, followed by western blotting with the indicated antibodies. ( b ) Effect of knockdown of vimentin in the surrounding cells on apical extrusion of Src-transformed cells. Data are mean±s.e. from three independent experiments. * P =0.0058 (Student’s t -test). ( c ) Effect of knockdown of vimentin in the surrounding cells on basal extension of Src-transformed cells. Data are mean±s.e. from three independent experiments. * P =0.013 (Student’s t -test). ( d ) Immunofluorescence images of vimentin (red) in the mix culture of normal and RasV12-transformed cells. RasV12-MDCK cells (stained with CMFDA, green) were mixed with normal MDCK cells. ( e ) Immunofluorescence images of keratin5+8 (red) in the mix culture of normal and RasV12-transformed cells. RasV12-MDCK cells (stained with CMFDA, green) were mixed with normal MDCK cells. Arrows indicate vimentin ( d ) or keratin5+8 ( e ) accumulation in normal MDCK cells at the interface with RasV12-MDCK cells. Scale bars, 10 μm ( d , e ). Full size image Filamin is a key regulator in the elimination of transformed cells We next examined spatial and functional relationship between filamin and vimentin. We observed that filamin and vimentin partially colocalized at the interface between normal and Src-transformed cells ( Fig. 6a ), consistent with the result of co-immunoprecipitation of filamin and vimentin ( Supplementary Fig. 1c ). When Src-transformed cells were surrounded by filamin A-knockdown cells, vimentin accumulation was significantly suppressed ( Fig. 6b ). In contrast, when Src-transformed cells were surrounded by vimentin-knockdown cells, filamin accumulation was not affected ( Fig. 6c ). These results suggest that filamin acts, at least partially, upstream of vimentin at the interface between normal and Src-transformed cells. Previous studies suggest that filamin acts upstream of vimentin during cell spreading and that protein kinase C-ε (PKC-ε) is involved in filamin-mediated vimentin phosphorylation that regulates dynamic reorganization of vimentin filaments [23] , [24] . We observed that PKC-ε was accumulated in normal cells but not in filamin-knockdown cells, at the interface with Src cells ( Fig. 6d ), suggesting that filamin regulates accumulation of PKC-ε. We also found that phosphorylated vimentin was colocalized with accumulated GFP-vimentin at the interface with Src-transformed cells ( Fig. 6e ), which was substantially suppressed by the treatment with PKC inhibitor bisindolylmaleimide (BIM)-I. BIM-I treatment also blocked apical extrusion of Src cells ( Fig. 6f ) and suppressed vimentin accumulation ( Fig. 6g ), but did not affect filamin accumulation ( Fig. 6h ). Collectively, these data suggest that PKC-ε is a potential regulator for filamin-regulated vimentin accumulation. 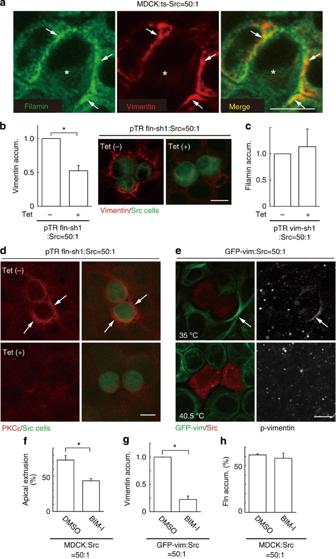Figure 6: Filamin acts as a key mediator in the interaction between normal and transformed epithelial cells. (a) Immunofluorescence images of filamin (green) and vimentin (red). Asterisks indicate the Src-transformed cell surrounded by normal cells. Arrows indicate colocalization of filamin and vimentin in the neighbouring normal cells at the interface with the Src-transformed cell. (b) Quantification of vimentin accumulation in filamin A-knockdown cells at the interface with Src-transformed cells. Representative images were shown on the right. Values are expressed as a ratio relative to tet (−). Data are mean±s.e. from three independent experiments. *P=0.0020 (Student’st-test). (c) Quantification of filamin accumulation in vimentin-knockdown cells at the interface with Src-transformed cells. Data are mean±s.e. from three independent experiments. Values are expressed as a ratio relative to tet (−). (d) Immunofluorescence images of PKC-ε (red) in the mix culture of MDCK pTR-filamin shRNA1 and ts-Src MDCK cells (green). Filamin shRNA1 expression was not induced (upper panels) or induced by tetracycline (lower panels). Arrows indicate the accumulation of PKC-ε in the surrounding cells at the interface with ts-Src MDCK cells. (e) Immunofluorescence images of phosphorylated vimentin (p-Ser38) in the mix culture of MDCK GFP-vimentin and ts-Src MDCK cells. Arrows indicate colocalization of phosphorylated-vimentin (white) and accumulated GFP-vimentin at the interface with Src-transformed cells (red). v-Src activation was induced at 35 °C (upper panels) or not induced at 40.5 °C (lower panels). Scale bars, 10 μm (a,b,d,e). (f) Effect of BIM-I on apical extrusion of Src-transformed cells. Data are mean±s.e. from three independent experiments. *P=0.0078 (Student’st-test). (g) Effect of BIM-I on vimentin accumulation at the interface with Src-transformed cells. Data are mean±s.e. from two independent experiments. Values are expressed as a ratio relative to dimethyl sulphoxide (DMSO). *P=0.0037 (Student’st-test). (h) Effect of BIM-I on filamin accumulation in the surrounding normal cells at the interface with Src-transformed cells. Data are mean±s.e. from two independent experiments. Figure 6: Filamin acts as a key mediator in the interaction between normal and transformed epithelial cells. ( a ) Immunofluorescence images of filamin (green) and vimentin (red). Asterisks indicate the Src-transformed cell surrounded by normal cells. Arrows indicate colocalization of filamin and vimentin in the neighbouring normal cells at the interface with the Src-transformed cell. ( b ) Quantification of vimentin accumulation in filamin A-knockdown cells at the interface with Src-transformed cells. Representative images were shown on the right. Values are expressed as a ratio relative to tet (−). Data are mean±s.e. from three independent experiments. * P =0.0020 (Student’s t -test). ( c ) Quantification of filamin accumulation in vimentin-knockdown cells at the interface with Src-transformed cells. Data are mean±s.e. from three independent experiments. Values are expressed as a ratio relative to tet (−). ( d ) Immunofluorescence images of PKC-ε (red) in the mix culture of MDCK pTR-filamin shRNA1 and ts-Src MDCK cells (green). Filamin shRNA1 expression was not induced (upper panels) or induced by tetracycline (lower panels). Arrows indicate the accumulation of PKC-ε in the surrounding cells at the interface with ts-Src MDCK cells. ( e ) Immunofluorescence images of phosphorylated vimentin (p-Ser38) in the mix culture of MDCK GFP-vimentin and ts-Src MDCK cells. Arrows indicate colocalization of phosphorylated-vimentin (white) and accumulated GFP-vimentin at the interface with Src-transformed cells (red). v-Src activation was induced at 35 °C (upper panels) or not induced at 40.5 °C (lower panels). Scale bars, 10 μm ( a , b , d , e ). ( f ) Effect of BIM-I on apical extrusion of Src-transformed cells. Data are mean±s.e. from three independent experiments. * P =0.0078 (Student’s t -test). ( g ) Effect of BIM-I on vimentin accumulation at the interface with Src-transformed cells. Data are mean±s.e. from two independent experiments. Values are expressed as a ratio relative to dimethyl sulphoxide (DMSO). * P =0.0037 (Student’s t -test). ( h ) Effect of BIM-I on filamin accumulation in the surrounding normal cells at the interface with Src-transformed cells. Data are mean±s.e. from two independent experiments. Full size image To explore the upstream regulators of filamin, we examined the effect of various inhibitors on filamin accumulation ( Supplementary Table 1 ). We found that Rho kinase inhibitor Y27632 significantly suppressed filamin accumulation in normal cells at the interface with RasV12- or Src-transformed cells ( Fig. 7a,b ). When RasV12- or Src-transformed cells were surrounded by cells overexpressing RhoGAP or a dominant negative mutant of Rho kinase, both apical extrusion and filamin accumulation were substantially suppressed ( Fig. 7c–j and Supplementary Fig. 10a,b ). Overexpression of a dominant negative form of myosin-II (myosin light chain (MLC)-AA) in normal cells surrounding Src-transformed cells did not affect apical extrusion or filamin accumulation ( Supplementary Fig. 10c–e ). These data indicate that in the surrounding normal cells the Rho/Rho kinase pathway regulates filamin accumulation in a myosin-II-independent manner. 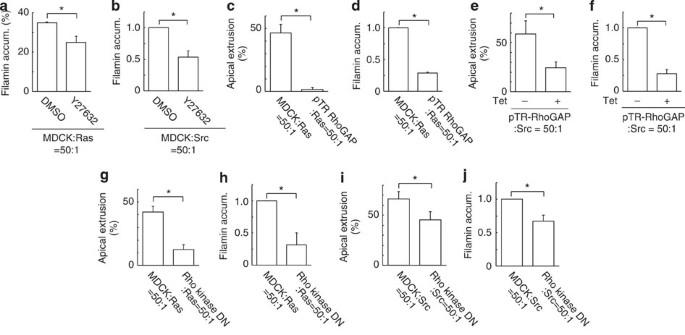Figure 7: The Rho-Rho kinase pathway in the surrounding normal cells is involved in filamin accumulation at the boundary with transformed cells. (a) Effect of Y27632 on filamin accumulation at the interface with RasV12-MDCK cells. Data are mean±s.e. from two independent experiments. *P=0.044 (Student’st-test ). (b) Effect of Y27632 on filamin accumulation at the interface with ts-Src MDCK cells. Data are mean±s.e. from three independent experiments. Values are expressed as a ratio relative to dimethyl sulphoxide (DMSO). *P=0.0045 (Student’st-test). (c,d) Effect of overexpression of RhoGAP in the surrounding cells on apical extrusion of RasV12-MDCK cells (c) or filamin accumulation at the interface with RasV12-MDCK cells (d). Data are mean±s.e. from two independent experiments. Values are expressed as a ratio relative to MDCK:Ras=50:1 (d). *P=0.011 (c), *P=2.8 × 10−4(d) (Student’st-test). (e,f) Effect of overexpression of RhoGAP in the surrounding cells on apical extrusion of ts-Src MDCK cells (e) or filamin accumulation at the interface with ts-Src MDCK cells (f). Data are mean±s.e. from three independent experiments. Values are expressed as a ratio relative to tet (−) (f). *P=0.041 (e), *P=2.0 × 10−4(f) (Student’st-test). (g,h) Effect of overexpression of a dominant negative mutant of Rho kinase in the surrounding cells on apical extrusion of RasV12-MDCK cells (g) or filamin accumulation at the interface with RasV12-MDCK cells (h). Data are mean±s.e. from three (g) or two (h) independent experiments. Values are expressed as a ratio relative to MDCK:Ras=50:1 (h). *P=0.0040 (g), *P=0.033 (h) (Student’st-test). (i,j) Effect of overexpression of a dominant negative mutant of Rho kinase in the surrounding cells on apical extrusion of ts-Src MDCK cells (i) or filamin accumulation at the interface with ts-Src MDCK cells (j). Data are mean±s.e. from five (i) or three (j) independent experiments. Values are expressed as a ratio relative to MDCK:Src=50:1 (j). *P=0.040 (i), *P=0.011 (j) (Student’st-test). Figure 7: The Rho-Rho kinase pathway in the surrounding normal cells is involved in filamin accumulation at the boundary with transformed cells. ( a ) Effect of Y27632 on filamin accumulation at the interface with RasV12-MDCK cells. Data are mean±s.e. from two independent experiments. * P =0.044 (Student’s t -test ). ( b ) Effect of Y27632 on filamin accumulation at the interface with ts-Src MDCK cells. Data are mean±s.e. from three independent experiments. Values are expressed as a ratio relative to dimethyl sulphoxide (DMSO). * P =0.0045 (Student’s t -test). ( c , d ) Effect of overexpression of RhoGAP in the surrounding cells on apical extrusion of RasV12-MDCK cells ( c ) or filamin accumulation at the interface with RasV12-MDCK cells ( d ). Data are mean±s.e. from two independent experiments. Values are expressed as a ratio relative to MDCK:Ras=50:1 ( d ). * P =0.011 ( c ), * P =2.8 × 10 −4 ( d ) (Student’s t -test). ( e , f ) Effect of overexpression of RhoGAP in the surrounding cells on apical extrusion of ts-Src MDCK cells ( e ) or filamin accumulation at the interface with ts-Src MDCK cells ( f ). Data are mean±s.e. from three independent experiments. Values are expressed as a ratio relative to tet (−) ( f ). * P =0.041 ( e ), * P =2.0 × 10 −4 ( f ) (Student’s t -test). ( g , h ) Effect of overexpression of a dominant negative mutant of Rho kinase in the surrounding cells on apical extrusion of RasV12-MDCK cells ( g ) or filamin accumulation at the interface with RasV12-MDCK cells ( h ). Data are mean±s.e. from three ( g ) or two ( h ) independent experiments. Values are expressed as a ratio relative to MDCK:Ras=50:1 ( h ). * P =0.0040 ( g ), * P =0.033 ( h ) (Student’s t -test). ( i , j ) Effect of overexpression of a dominant negative mutant of Rho kinase in the surrounding cells on apical extrusion of ts-Src MDCK cells ( i ) or filamin accumulation at the interface with ts-Src MDCK cells ( j ). Data are mean±s.e. from five ( i ) or three ( j ) independent experiments. Values are expressed as a ratio relative to MDCK:Src=50:1 ( j ). * P =0.040 ( i ), * P =0.011 ( j ) (Student’s t -test). Full size image We previously reported that myosin-II was activated in Src- or Ras-transformed cells when surrounded by normal cells and that addition of myosin-II inhibitor blebbistatin or coexpression of MLC-AA in the transformed cells substantially suppressed their apical extrusion [8] , [11] . We found that addition of blebbistatin significantly suppressed filamin accumulation in normal cells at the interface with Src-transformed cells ( Fig. 8a ). In addition, expression of MLC-AA in Src- or Ras-transformed cells significantly suppressed filamin accumulation in the surrounding normal cells ( Fig. 8b–d ). These data suggest that the activation of myosin-II in transformed cells influences localization and function of filamin in the neighbouring normal cells. It has been reported that myosin-II activity affects various cellular mechanical properties [25] , [26] . Thus, we next performed atomic force microscopic (AFM) analyses and found that Ras-transformed cells had higher elasticity than normal cells, and coexpression of MLC-AA significantly suppressed it ( Supplementary Fig. 11 ) [8] , indicating that enhanced myosin-II activity leads to increased cellular elasticity in the transformed cells. Together with the previous study showing that filamin acts as mechanosensor/transducer [17] , these data support the notion that normal cells sense and respond to mechanical environments modulated by myosin-II-driven forces in the neighbouring transformed cells, and that filamin plays a crucial role in this process. 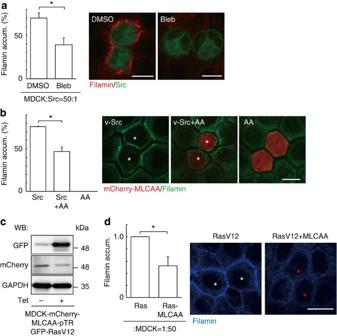Figure 8: Myosin-II activity in transformed cells regulates filamin accumulation in the surrounding normal cells. (a) Effect of blebbistatin on filamin accumulation in the surrounding normal cells at the interface with Src-transformed cells. Data are mean±s.e. from three independent experiments. *P=0.024 (Student’st-test). (b) Effect of MLC-AA expression in v-Src-expressing cells on filamin accumulation in the surrounding normal cells. v-Src and/or mCherry-tagged MLC-AA were transiently transfected in MDCK cells. v-Src-transfected cells were identified by immunofluorescence using anti-pY418-Src antibody. Asterisks indicate v-Src-expressing cells. AA; MLC-AA. Data are mean±s.e. from three independent experiments. *P=0.0028 (Student’st-test). (c) Establishment of MDCK-pTR GFP-RasV12 cells stably expressing mCherry-MLC-AA. The expression of GFP-RasV12 was not induced or induced for 24 h by tetracycline, followed by western blotting with the indicated antibodies. (d) Effect of MLC-AA-coexpression in RasV12-transformed cells on filamin accumulation in the surrounding normal cells. Cells were stained with anti-filamin antibody (blue). White and red asterisks indicate RasV12- and RasV12+MLC-AA-expressing cells, respectively. Data are mean±s.e. from three independent experiments. Values are expressed as a ratio relative to RasV12-expressing cells. *P=0.017 (Student’st-test). Representative images were shown on the right (a,b,d). Scale bars, 10 μm (a,b,d). Figure 8: Myosin-II activity in transformed cells regulates filamin accumulation in the surrounding normal cells. ( a ) Effect of blebbistatin on filamin accumulation in the surrounding normal cells at the interface with Src-transformed cells. Data are mean±s.e. from three independent experiments. * P =0.024 (Student’s t -test). ( b ) Effect of MLC-AA expression in v-Src-expressing cells on filamin accumulation in the surrounding normal cells. v-Src and/or mCherry-tagged MLC-AA were transiently transfected in MDCK cells. v-Src-transfected cells were identified by immunofluorescence using anti-pY418-Src antibody. Asterisks indicate v-Src-expressing cells. AA; MLC-AA. Data are mean±s.e. from three independent experiments. * P =0.0028 (Student’s t -test). ( c ) Establishment of MDCK-pTR GFP-RasV12 cells stably expressing mCherry-MLC-AA. The expression of GFP-RasV12 was not induced or induced for 24 h by tetracycline, followed by western blotting with the indicated antibodies. ( d ) Effect of MLC-AA-coexpression in RasV12-transformed cells on filamin accumulation in the surrounding normal cells. Cells were stained with anti-filamin antibody (blue). White and red asterisks indicate RasV12- and RasV12+MLC-AA-expressing cells, respectively. Data are mean±s.e. from three independent experiments. Values are expressed as a ratio relative to RasV12-expressing cells. * P =0.017 (Student’s t -test). Representative images were shown on the right ( a , b , d ). Scale bars, 10 μm ( a , b , d ). Full size image In this study, we demonstrate the molecular mechanisms whereby normal epithelial cells actively eliminate neighbouring transformed cells from the epithelium. We present several data indicating that filamin is a key mediator in the interaction between normal and transformed epithelial cells. First, in mammalian cultured cells, filamin accumulates in normal epithelial cells at the interface with Src- or Ras-transformed cells. Knockdown of filamin in normal epithelial cells profoundly suppresses apical extrusion of the neighbouring transformed cells. Second, in the EVL epithelium of zebrafish embryos, filamin is accumulated around v-Src-expressing cells, and knockdown of filamin significantly diminishes their apical extrusion. Third, the Rho/Rho kinase pathway regulates filamin accumulation and filamin acts upstream of vimentin filaments that dynamically react against transformed cells. These data indicate that filamin plays a vital role in apical extrusion of transformed cells. Laser ablation experiments revealed that pulling forces are exerted on the interface between normal and transformed cells ( Supplementary Fig. 12 and Supplementary Movies 4–6 ). When transformed cells are surrounded by normal cells, myosin-II activity is enhanced and the transformed cells become round and tall, suggesting the elevated tensile forces within the transformed cells [8] , [11] . Furthermore, reduction of myosin-II activity in the transformed cells diminishes these morphological changes [8] . Collectively, the pulling forces at the interface are likely to be mediated by enhanced myosin-II activity in the transformed cells, which would physically drive the apical extrusion process. In addition, vimentin filaments in the neighbouring normal cells may also play a role in this process. When Src cells are surrounded by vimentin-knockdown cells, formation of p-MLC-enriched basal protrusions is significantly promoted, and instead p-MLC is downregulated along the lateral membranes ( Supplementary Fig. 8d ); thus, the presence of vimentin filaments in normal cells substantially influences the localization of p-MLC in the neighbouring transformed cells. The molecular mechanism underlying this process is not clear at present, which needs to be elucidated in future studies. Within the epithelia of Drosophila and mammals, normal and transformed cells have been shown to compete with each other for survival. Either of them are extruded from the epithelium or undergo apoptosis, while the other proliferate and fill the vacant spaces [9] , [10] , [27] , [28] , [29] . These phenomena potentially reflect the events occurring at the initial stage of carcinogenesis; however, the molecular mechanisms, especially for cell extrusion, are still largely unknown. Previous studies showed that when Ras- or Src-transformed cells are surrounded by normal cells, various proteins such as myosin-II, MAPK, Cdc42 and N-WASP are upregulated in transformed cells, leading to their apical extrusion [8] , [11] , [30] . In addition, upregulation of MAPK and matrix metalloproteinases in ErbB2-overexpressing cells is involved in their apical translocation [12] . In the imaginal disc epithelium of Drosophila , activity of Rho1 and JNK in Src-activated cells is engaged in their extrusion [7] , [31] . These results indicate that multiple signalling pathways modulated in the transformed cells are implicated in their elimination from epithelia. However, it remained elusive whether and how normal cells actively influence the fate of neighbouring transformed cells. Here we show that filamin is a key regulator in normal epithelial cells to eliminate transformed cells. This is the first report demonstrating the molecular mechanism whereby normal epithelial cells play an active role in apical extrusion of transformed cells ( Fig. 9 ). Our results imply a notion that at the early stage of carcinogenesis, normal epithelial cells act as ‘immunity’ against transformed cells; here we name this process as EDAC (epithelial defence against cancer). By further developing this new research field, we would create a novel type of cancer treatment: eradication of transformed cells by enhancing a defensive force of neighbouring normal epithelial cells. 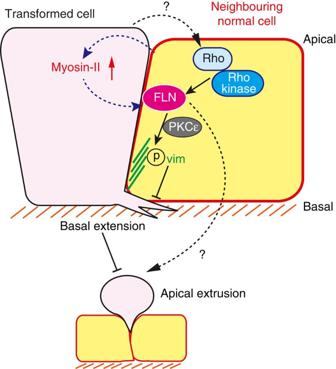Figure 9: Molecular mechanisms of EDAC (Epithelial Defence Against Cancer). A schematic model of molecular mechanisms for the defensive force of the neighbouring normal cells against transformed cells. When transformed cells are surrounded by normal epithelial cells, myosin-II activity is upregulated in the transformed cells, which in turn induces filamin (FLN) accumulation in the normal cells at the interface in a Rho/Rho kinase-dependent manner. Accumulated filamin regulates dynamic movement of vimentin (vim) through its phosphorylation via PKC-ε. Holding arm-like vimentin filaments in normal cells generate contractile forces at the interface that prevent the neighbouring transformed cells from forming basal extensions, thereby promoting their apical extrusion from the epithelial monolayer. Figure 9: Molecular mechanisms of EDAC (Epithelial Defence Against Cancer). A schematic model of molecular mechanisms for the defensive force of the neighbouring normal cells against transformed cells. When transformed cells are surrounded by normal epithelial cells, myosin-II activity is upregulated in the transformed cells, which in turn induces filamin (FLN) accumulation in the normal cells at the interface in a Rho/Rho kinase-dependent manner. Accumulated filamin regulates dynamic movement of vimentin (vim) through its phosphorylation via PKC-ε. Holding arm-like vimentin filaments in normal cells generate contractile forces at the interface that prevent the neighbouring transformed cells from forming basal extensions, thereby promoting their apical extrusion from the epithelial monolayer. Full size image Antibodies, plasmids and materials Mouse anti-phospho-tyrosine (clone 4G10; 05-1050), mouse anti-actin (MAB1501R), mouse anti-myc-tag (clone 4A6;05-724), mouse anti-GAPDH (MAB374) and rabbit anti-integrin β3 (04-1060) antibodies were from Merck Millipore. Mouse anti-phospho-tyrosine (P-Tyr-100; 9411), rabbit anti-vimentin (5741) and rabbit anti-phospho-MLC 2 (Thr18/Ser19; 3674) antibodies were from Cell Signaling Technology. As to anti-phospho-tyrosine antibodies, clone 4G10 was used for western blotting and a mixture of the two antibodies was used for immunoprecipitation. Mouse anti-vimentin (clone V9; V6389) and mouse anti-filamin (F6682) antibodies were from Sigma-Aldrich. Mouse anti-integrin β1 (610467), mouse anti-E-cadherin (610182), mouse anti-N-cadherin (610920) and mouse anti-β-catenin (610153) antibodies were from BD Biosciences. Rabbit anti-phospho-vimentin (Ser38; ab52942) and mouse anti-PKC-ε (ab114034) antibodies were from Abcam. Mouse anti-GFP (11814460001) antibody was from Roche Diagnostics. Rabbit anti-pY418-Src (44660G) antibody was from Life Technologies. Mouse anti-mCherry (632543) antibody was from Clontech. Mouse anti-keratin K5/K8 (65131) antibody was from PROGEN Biotechnik GmbH. For Fig. 6a , Alexa-Fluor-568-conjugated anti-vimentin antibody was prepared using Zenon Mouse IgG Labeling Kit (Life Technologies) according to the manufacturer’s instructions. Alexa-Fluor-488-, -568- or -647-conjugated phalloidin (Life Technologies) was used at 1.0 U ml −1 . Alexa-Fluor-488-, -568- and -647-conjugated secondary antibodies were from Life Technologies. Hoechst 33342 (Life Technologies) was used at a dilution of 1:5,000. For immunofluorescence, all primary antibodies were used at 1:100, except for anti-PKC-ε and anti-phospho-MLC 2 antibodies that were used at 1:50, and all secondary antibodies were used at 1:200. To construct pEGFP-N1-vimentin, the complementary DNA of human vimentin was obtained from Addgene and inserted into pEGFP-N1. To construct pcDNA/TO/GFP-MLC-AA, the cDNA of MLC-AA was amplified from pEGFP-N1-MLC-AA (gift from H. Hosoya) by PCR and inserted into the Xho I/ Eco RI site of pcDNA/TO/GFP [32] . To construct pmCherry-N1-MLC-AA, the cDNA of MLC-AA was inserted into the Eco RI/ Kpn I site of pmCherry-N1 (gift from R. Y. Tsien). pcDNA/TO/Cherry-p50RhoGAP catalytic domain was as previously described [8] . pEF-BOS-myc-Rho kinase RB/PH (TT) (a dominant negative mutant) was provided by K. Kaibuchi. Type-I collagen (Cellmatrix Type I-A) was obtained from Nitta Gelatin and was neutralized on ice to a final concentration of 2 mg ml −1 according to the manufacturer’s instructions. To fluorescently stain living MDCK, ts-Src MDCK or MDCK-pTR GFP-RasV12 cells, CMTPX (red dye) or CMFDA (green dye) (Life Technologies) was used according to the manufacturer’s instructions. The following inhibitors, BIM-I (10 μM), CK666 (100 μM), (S)-(-)-blebbistatin (30 μM), KT5720 (4 μM), IPA-3 (40 μM), Smifh2 (25 μM) and Y27632 (20 μM) were from Calbiochem. U0126 (40 μM) was from Promega. Cytochalasin D (4 μM) was from Sigma-Aldrich. Cell culture MDCK and ts-Src MDCK cells were from W. Birchmeier [19] and were cultured as previously described [8] , [11] . MDCK-pTR GFP-RasV12 cells were cultured in DMEM containing 10% FCS (tetracycline free), penicillin/streptomycin, 5 μg ml −1 of blasticidin (Invivogen) and 400 μg ml −1 of zeocin (Invivogen) [8] . MDCK cells stably expressing yellow fluorescent protein (YFP)-actin (gift from J. Rosenblatt) were cultured as MDCK cells, except that 800 μg ml −1 of G418 (Calbiochem) was added to the medium. To establish MDCK cells stably expressing GFP-vimentin or myc-Rho kinase RB/PH (TT), MDCK cells were transfected with pEGFP-N1-vimentin or pEF-BOS-myc-Rho kinase RB/PH (TT) using Lipofectamine 2000 (Life Technologies) according to the manufacturer’s instructions, followed by selection in medium containing 800 μg ml −1 of G418. For establishing cell lines stably expressing myc-Rho kinase RB/PH (TT), pcDNA-FLAG was co-transfected to induce neomycin resistance. MDCK cells stably expressing filamin A short hairpin RNA (shRNA) or vimentin shRNA in a tetracycline-inducible manner were established as follows; filamin A shRNA oligonucleotides (filamin A shRNA-1: 5′-GATCCCCGCTGGAGTGCCAGCTGAATTTCAAGAGAATTCAGCTGGCACTCCAGCTTTTTC-3′ and 5′-TCGAGAAAAAGCTGGAGTGCCAGCTGAATTCTCTTGAA ATTCAGCTGGCACTCCAGCGGG-3′ or filamin A shRNA-2: 5′-GATCCCC GCCTAGCAAGGTGAAGGCGTTCAAGAGACGCCTTCACCTTGCTAGGCTTTTTC-3′ and 5′-TCGAGAAAAAGCCTAGCAAGGTGAAGGCGTCTCTTGAA CGCCTTCACCTTGCTAGGC GGG-3′), or vimentin shRNA oligonucleotides (vimentin shRNA-1: 5′-GATCCCCGCTGCTAACTACCAAGACATTCAAGAGATGTCTTGGTAGTTAGCAGCTTTTTC-3′ and 5′-TCGAGAAAAAGCTGCTAACTACCAAGACATCTCTTGAATGTCTTGGTAGTTAGCAGCGGG-3′, or vimentin shRNA-2: 5′-GATCCCCGATGGCTCTCGACATTGAGTTCAAGAGACTCAATGTCGAGAGCCATCTTTTTC-3′ and 5′-TCGAGAAAAAGATGGCTCTCGACATTGAGTCTCTTGAACTCAATGTCGAGAGCCATCGGG-3′) were cloned into the Bgl II and Xho I site of pSUPERIOR.neo+gfp (Oligoengine). MDCK-pTR cells [8] were transfected with pSUPERIOR.neo+gfp filamin A shRNA or vimentin shRNA using Lipofectamine 2000, followed by selection in medium containing 5 μg ml −1 of blasticidin and 800 μg ml −1 of G418. To establish MDCK cells stably expressing GFP-MLC-AA or mCherry-p50RhoGAP catalytic domain in a tetracycline-inducible manner, MDCK-pTR cells were transfected with pcDNA/TO/GFP-MLC-AA or pcDNA/TO/mCherry-p50RhoGAP catalytic domain as described above, followed by selection in medium containing 5 μg ml −1 of blasticidin and 400 μg ml −1 of zeocin. To establish MDCK-pTR GFP-RasV12 cells stably expressing mCherry-MLC-AA, MDCK-pTR GFP-RasV12 cells were transfected with pmCherry-N1-MLC-AA as described above, followed by selection in medium containing 5 μg ml −1 of blasticidin, 400 μg ml −1 of zeocin and 800 μg ml −1 of G418. For tetracycline-inducible MDCK cell lines, 2 μg ml −1 of tetracycline (Sigma-Aldrich) was used to induce expression of proteins or shRNAs. All inhibitors were added at the beginning of the experiments for 12–24 h incubation, except that Cytochalasin D was added for 1 h before fixation. BIM-I was replaced every 12 h for 24 h. For Fig. 8b , MDCK cells were seeded on collagen-coated coverslips in 35-mm dishes (Greiner-Bio-One) at a density of 1.0 × 10 6 cells and incubated for 24 h. Cells were then transiently transfected with pSG-v-Src [19] and/or pmCherry-N1-MLC-AA using Lipofectamine 2000 (Life Technologies), and were analysed after 18 h. For Figs 5b,c and 6c , and Supplementary Fig. 8c,d , MDCK-pTR vimentin-shRNA1 or -shRNA2 cells were incubated with tetracycline for 72 h before induction of v-Src activation. For Figs 2i,j and 6b,d , and Supplementary Fig. 3b , to induce sufficient knockdown of filamin A protein, MDCK-pTR filamin A-shRNA1 cells were incubated with tetracycline for 48 h before induction of v-Src activation or RasV12 expression. Similarly, for Supplementary Fig. 3d , MDCK-pTR filamin A-shRNA2 cells were incubated with tetracycline for 72 h before induction of v-Src activation. Immunoprecipitation and western blotting For immunoprecipitation, MDCK and ts-Src MDCK cells were trypsinized and plated at a density of 1.6 × 10 7 cells in 14.5-cm dishes (Greiner-Bio-One) and cultured at 40.5 °C for 9 h until a monolayer was formed. Src activation was then induced at 35 °C for 14 h. Cells were washed with ice-cold PBS containing 1 mM Na 3 VO 4 and lysed for 30 min in Triton X-100 lysis buffer (20 mM Tris-HCl, pH 7.5, 150 mM NaCl, 1% Triton X-100, 1 mM Na 3 VO 4 and 10 mM NaF) containing 5 μg ml −1 leupeptin, 1 mM phenylmethylsulphonyl fluoride and 7.2 trypsin inhibitor units of aprotinin. After centrifugation at 21,500 g for 10 min, the supernatants were subjected to immunoprecipitation for 1 h with Dynabeads Protein G (Life Technologies) conjugated with a mixture of anti-phospho-tyrosine antibodies (clone 4G10 and P-Tyr-100; 5 μg each). Immunoprecipitated proteins were subjected to SDS–PAGE analysis, followed by SYPRO Ruby protein gel staining (Life Technologies) or western blotting with the indicated antibodies. SYPRO Ruby protein staining was performed according to the manufacturer’s instructions. Western blotting was performed as previously described [33] . Primary antibodies were used at 1:1,000, except anti-GAPDH at 1:2,000. Stained gels and western blotting data were analysed using ImageQuant LAS4010 (GE Healthcare). Time-lapse microscopy and immunofluorescence For time-lapse analyses, MDCK or ts-Src MDCK cells were fluorescently labelled, mixed with MDCK cells stably expressing GFP-vimentin at a ratio of 1:50 and seeded on the collagen matrix as previously described [8] , [11] . The mixture of cells was incubated at 40.5 °C for 8–12 h until a monolayer was formed, and was observed at 35 °C by Olympus IX81 microscope with the FV1000 system equipped with Z focus drift compensating system, followed by analyses using Olympus FV10-ASW or Volocity software (Improvision). For immunofluorescence, MDCK-pTR GFP-RasV12 or ts-Src MDCK cells were stained with CMTPX or CMFDA, mixed with the indicated non-stained cells at a ratio of 1:50, and cultured on the collagen matrix as previously described [8] . For analyses of ts-Src MDCK cells, the mixture of cells was incubated for 8–12 h at 40.5 °C until a monolayer was formed, followed by v-Src activation at 35 °C for 12 h, except for analyses of apical extrusions that were examined after 24 h of v-Src activation and for immunofluorescence of PKC-ε that were examined after 10 h of v-Src activation. For analyses of MDCK-pTR GFP-RasV12 cells, the mixture of cells was incubated for 8–12 h, followed by tetracycline treatment for 16 h, except for analyses of apical extrusions that were examined after 24 h of tetracycline treatment. Cells were fixed in methanol for 2.5 min at −20 °C, except that for Figs 4c and 6d , and Supplementary Figs 2a,b,d, 7b,c, 8d and 9b , cells were fixed with 4% paraformaldehyde (PFA) in PBS and permeabilized as previously described [11] . Immunofluorescence images were analysed by Leica TCS SPE confocal microscope system and Leica Application Suite, or Olympus FV1000 system and Olympus FV10-ASW software. Images were quantified by MetaMorph software (Molecular Devices). Electron microscopy The mixtures of ts-Src MDCK cells and MDCK or MDCK GFP-vimentin cells were prepared and cultured in collagen gel-coated, photo-etched grid-glass bottom dishes (MatTek Corporation) as described in ‘Time-lapse microscopy and immunofluorescence’. Briefly, after 12 h of v-Src activation, cells were fixed primarily in 4% PFA before target cells were identified and documented by fluorescence and differential interference contrast (DIC) imaging. Cells were then fixed in PFA/glutaraldehyde, secondarily fixed with osmium tetroxide/potassium ferricyanide before being dehydrated and embedded in EPON. Serial ultrathin sections were stained with lead citrate before being visualized and imaged in a Tecnai Spirit G2 120 kV TEM (FEI) coupled to a Morada charge-coupled device camera (Olympus SIS). Protein identification by mass spectrometry Protein bands were excised from the gel, and the protein was identified by peptide mass fingerprinting and post-source decay tandem mass spectrometry (MS/MS) analysis. Briefly, protein bands were digested in-gel by trypsin gold (Promega) after reductive S-alkylation with dithiothreitol and iodoacetamide. After incubation at 37 °C for 12 h, tryptic peptides were purified by ZipTip mC18 (Millipore). High-purity α-cyano-4-hydroxycinnamic acid (Shimadzu GLC) was used as matrix-assisted laser desorption/ionization matrix. Mass spectrometric analysis was performed by AXIMA Performance matrix-assisted laser desorption/ionization–time of flight MS (Shimadzu Corporation). The acquisition mass range was 700–4,000 Da. Mass spectrometer was first externally calibrated by angiotensin II ( m/z 1046.54) and ACTH fragment 18–39 ( m/z 2465.20), and each result was internally calibrated by tryptic autolysis fragment ( m/z 842.51 and 2211.10). The peak processing of peptide mass spectra and MS/MS ion selection were analysed by Launchpad version 2.9.1 (Shimadzu) and protein was identified against NCBI non-redundant canis familiaris database (2011_11, 16,245,521 sequence entries) on Mascot Server version 2.3 (Matrix Science), up to one missed cleavage, peptide tolerance of 0.2 Da, fixed modifications of cysteine carbamydomethylation and variable modifications of methionine oxidation. MOlecular Weight SEarch (MOWSE) scores of mass fingerprinting above 56 were considered significant ( P <0.05) and ion scores of MS/MS above 28 were indicated identity or extensive homology ( P <0.05). Data analyses For data analyses, one-tailed Student’s t -tests were used to determine P -values, except in Fig. 4e , where two-tailed Fisher’s exact test was used, and Supplementary Fig. 12b , where Welch’s t -test was used. For quantification of apical extrusion or immunofluorescence intensity of Src- or RasV12-transformed cells, 1–3 Src-transformed cells or 2–8 RasV12-transformed cells that were surrounded by the indicated cells were analysed. For ts-Src MDCK cells, more than 50 cells were analysed for each experimental condition. For RasV12-MDCK cells, more than 50 cells were analysed for filamin accumulation or more than 120 cells were analysed for apical extrusion, except for Fig. 2j , where the number of RasV12-MDCK cell colonies in which the majority ( ⩾ 75%) of RasV12 cells were apically extruded was counted ( n =60 colonies from two independent experiments). Filamin accumulation in the surrounding cells at the interface with Src- or RasV12-transformed cells was quantified per transformed cell. Apical extrusion was analysed by confocal microscopy. For Fig. 2d , n =107 for Src-transformed MDCK cells and n =63 for MDCK cells from two to five independent experiments. For Fig. 5c , to analyse basal extensions of Src-transformed cells, the number of p-MLC-enriched basal extensions below neighbouring cells were quantified. For Fig. 6b , to quantify diminished vimentin accumulation in filamin A-knockdown cells, immunofluorescence intensity of two vimentin-accumulated spots (36 pixels each) per surrounded Src-transformed cell was quantified. When the average of the intensity from the two spots was higher than the average of that in all tetracycline-negative images, the cell was counted as vimentin accumulation positive. Vimentin accumulation around more than 35 Src cells was quantified in each experiment; tet (−), n =134; tet (+), n =145 from three independent experiments. For Fig. 6c , filamin accumulation in vimentin-knockdown cells was analysed in a similar way as described above, except that two filamin-accumulated spots (16 pixels each) were analysed; tet (−), n =146; tet (+), n =124 from three independent experiments. For Supplementary Fig. 2c , the fluorescence intensity of YFP-actin in MDCK YFP-actin cells at the interface with normal or Src-transformed MDCK cells was analysed. For each surrounded normal or Src-transformed cell, fluorescence intensity of 4 spots (48 pixels each) in MDCK YFP-actin cells was quantified. More than 20 normal or Src-transformed cells were analysed in each experiment. YFP-actin:MDCK=50:1, n =69; YFP-actin:Src=50:1, n =82 from three independent experiments. For Fig. 3b , 275 cells from 10 embryos for control morpholino oligonucleotide (MO) and 219 cells from 9 embryos for filamin MO1 were analysed. For Fig. 3c , 417 cells from 12 embryos for control MO+GFP, 326 cells from 10 embryos for filamin MO1+GFP and 449 cells from 12 embryos for filamin MO1+GFP-filamin were analysed. For Supplementary Fig. 4b , 478 cells from 12 embryos for control MO and 391 cells from 12 embryos for splice MO2 were analysed. Transgenic lines and confocal imaging of zebrafish embryos To generate an EVL-specific tamoxifen-inducible Gal4-driver line, we replaced the Gal4 sequence of pBR-Tol2-krt18:Gal4 (ref. 11 ) with a fusion protein of the fish-optimized Gal4 KalTA4 (ref. 34 ) and ERT2 (gift from J. Brickman), KalTA4-ERT2. We generated a UAS:GFP-filamin line by placing GFP-tagged human filamin downstream of five copies of the UAS sequence (5 × UAS) [35] . The cDNA of human filamin A was obtained from DsRed2-filamin A (gift from M. Ikebe). The transgenic lines were generated using the Tol2 system [36] . We used the UAS:GAP43-GFP line [11] as a negative control. To visualize cells expressing v-Src, we employed a membrane-Cherry-tagged version of v-Src through the self-cleaving 2A sequence under the control of 5 × UAS [11] . Embryos were injected with the v-Src construct (10–20 pg) and Tol2 RNA (20 pg) into the cell at one-cell stage, and treated with 0.5 μM 4-hydroxy tamoxifen (Sigma H7904, a stock of 5 mM in ethanol) at 60% epiboly. The embryos were fixed in 4% PFA at 3-4 h after induction and were mounted in 1% low-melting agarose for confocal analyses. Confocal images were taken using a × 40 water-immersion lens on Leica DM2500 microscope with the TCS SPE system, and were analysed using the Volocity software (Perkin-Elmer). For knockdown experiments in zebrafish, we used two anti-sense MOs against filamin A gene: 5′-CGGGTCTCCTGCACTAATTCGCTGT-3′ (translational-blocking MO1) and 5′-ACCTGCACAGCAGAGAGCAATACCC-3′ (splice-blocking MO2). The splice MO2 was designed against Exon5, and was validated by RT–PCR for the presence of an aberrant splice form. We used a standard control MO from Gene Tools: 5′-CCTCTTACCTCAGTTACAATTTATA-3′. The MOs (8 ng) were injected into the yolk at the two-cell stage following injection of the v-Src construct. Atomic force microscopy A commercial AFM (MFP-3D, Asylum Research) with a rectangular cantilever (BL-AC40TS-C2, ~0.1 N m −1 ; Olympus) was used to examine the rheology of MDCK, RasV12-MDCK and RasV12-MLC-AA-MDCK cells. The AFM was mounted on an inverted optical microscope (TE-2000E, Nikon). A colloidal silica bead with a radius R of ~2.5 μm (Funakoshi) was attached to the apex of the tip with epoxy [37] . Before cell experiments, the spring constant of the cantilever was determined using a built-in thermal fluctuation procedure. For force modulation measurements, the cells around cel–cell contact sites were indented for ~30 s at an initial loading force of <650 pN. During indentation, a reference signal voltage containing several sinusoidal oscillations in the frequency range of f =5−100 Hz with an amplitude of 10 nm was applied to a z axis piezo actuator to move the cantilever in the direction normal to the sample surface. The amplitude and phase shift of the cantilever displacement with respect to the reference signal were measured using a digital lock-in amplifier (7260, SEIKO EG&G Co.). The complex shear modulus G* of cells was estimated according to previous procedures [37] , [38] . The storage G ′ and loss G ′′ moduli of single cells as a function of f were fitted to the power-law structural damping model with additional Newtonian viscosity [39] , which is given by Here, G 0 is a scale factor of the modulus at a frequency scale factor f 0 , which was arbitrarily set to 1 Hz. α is the power-law exponent. The g ( α ) is Γ(1− α ) cos( πα /2) where Γ denotes the γ -function. The hysteresivity η ( α ) is equivalent to tan( πα /2) and μ is the Newtonian viscous damping coefficient. G 0 exhibits a log-normal distribution and is positively correlated with the apparent Young’s modulus by AFM force curve measurements [37] . If α approaches zero, the cell is perfectly elastic. If α approaches unity, the cell follows the Newton’s law of viscous deformation [39] . The power-law rheological parameters of ln G 0 , α and μ of single cells estimated from equation (1) are shown in Supplementary Fig. 11 . The significant difference of those parameters among types of cells shown in Supplementary Fig. 11 remained unchanged even measured at the centre of cells. Laser ablation The mixtures of the indicated cells were seeded on collagen gel-coated glass-bottom dish and incubated as described in ‘Time-Lapse Microscopy and Immunofluorescence’. A 2-photon laser tuned to the 880 nm wavelength (Chameleon, Coherent) irradiated an inner region of the cell (~10 μm 2 ). The duration of the stimulus was 100 ms with an approximate power of 115 mW at the surface of the objective lens. In parallel with the ablation, images were acquired at 2 s intervals on an inverted multi-photon microscope (A1MP, Nikon) equipped with a Nikon × 40/NA1.15 Apo LWD water-immersion objective. For measuring mechanical stress in vimentin filaments, a 2-photon laser was used in point-scan mode (0.062 μm per pixel). The duration of the stimulus was 30 ms with an approximate power of 105 mW. Other settings were same as the cell ablation experiment. Data were analysed by using ImageJ. For Supplementary Fig. 9a , recoil velocity was calculated by measuring the distance between severed ends of laser-irradiated GFP-vimentin filaments at 0 and 18 s after laser irradiation. Eleven areas where GFP-vimentin was accumulated around ts-Src MDCK cells were analysed. How to cite this article: Kajita, M. et al . Filamin acts as a key regulator in epithelial defence against transformed cells. Nat. Commun. 5:4428 doi: 10.1038/ncomms5428 (2014).